IRX2 regulates angiotensin II-induced cardiac fibrosis by transcriptionally activating EGR1 in male mice Cardiac fibrosis is a common feature of chronic heart failure. Iroquois homeobox (IRX) family of transcription factors plays important roles in heart development; however, the role of IRX2 in cardiac fibrosis has not been clarified. Here we report that IRX2 expression is significantly upregulated in the fibrotic hearts. Increased IRX2 expression is mainly derived from cardiac fibroblast (CF) during the angiotensin II (Ang II)-induced fibrotic response. Using two CF-specific Irx2 -knockout mouse models, we show that deletion of Irx2 in CFs protect against pathological fibrotic remodelling and improve cardiac function in male mice. In contrast, Irx2 gain of function in CFs exaggerate fibrotic remodelling. Mechanistically, we find that IRX2 directly binds to the promoter of the early growth response factor 1 (EGR1) and subsequently initiates the transcription of several fibrosis-related genes. Our study provides evidence that IRX2 regulates the EGR1 pathway upon Ang II stimulation and drives cardiac fibrosis. Sustained cardiac stress results in excessive production of extracellular matrix components, causing cardiac fibrosis. Cardiac fibrosis can increase the stiffness of the left ventricle, disrupt cardiac conduction, and impair systolic and diastolic function [1] , [2] , [3] . The presence of fibrosis has been independently associated with cardiovascular mortality and all-cause mortality [4] . Currently, no evidence-based therapies show significant efficacy against fibrotic diseases, largely because the mechanisms of cardiac fibrosis are unclear. Moreover, our knowledge on the mechanisms of cardiac fibrosis is predominantly derived from experiments performed in cell culture systems or genetic mice with cardiomyocyte-specific manipulation [5] . Upon fibrogenic stimulation, quiescent cardiac fibroblasts (CFs) proliferate and differentiate into myofibroblasts, which express the highly contractile protein α-smooth muscle actin (α-SMA) [6] . Several growth factors and cytokines, such as transforming growth factor-β (TGF-β), angiotensin II (Ang II), platelet-derived growth factor (PDGF), fibroblast growth factor (FGF), and bone morphogenetic protein (BMP), are key driving forces culminating in the cardiac fibrotic response [7] . These growth factors and cytokines directly bind to their receptors and thus trigger the activation of downstream effector proteins, such as Smad3, to amplify the fibrotic response [7] . Increased knowledge of molecules that regulate multiple pro-fibrotic pathways may be translated into gene-based therapies for the treatment of cardiac fibrosis. Iroquois homeobox (IRX) genes were first identified in Drosophila melanogaster , and this family includes six homeoproteins, named IRX1-IRX6 [8] . During neurogenesis, Xiro (the Xenopus analogue of a human IRX member) functions as a repressor of BMP-4 after activation by the Wnt signalling pathway [9] . All six members display specific expression patterns in the heart and play key roles in heart development and function [10] , [11] . Specifically, IRX4 regulates chamber-specific gene expression in the developing heart, while IRX5 establishes the mouse cardiac ventricular repolarization gradient [10] , [11] . IRX2 has been shown to be induced by TGF-β [12] and FGF8 during chick hindlimb development [13] and to be regulated by sex-determining region Y box 9 (SOX9) [12] , which is a master regulator of cardiac fibrosis [14] . IRX2 was found to be increased in a mouse model of dilated cardiomyopathy (DCM) [15] , and could be activated by mitogen-activated protein kinases [13] . Despite the strong expression of IRX2 in the heart, its effects in diseased hearts, especially in CF activation and fibrotic remodelling, have not been investigated. Here, we identified IRX2 as a CF-enriched transcription factor that promotes the development of pathological cardiac fibrosis by transcriptionally activating growth response factor 1 (EGR1). To the best of our knowledge, this is the first report describing a causative role for IRX2 in fibrotic remodelling. IRX2 expression is upregulated in a murine model of cardiac fibrosis and in human fibrotic hearts To detect alterations in IRXs during the fibrotic process, isolated mouse CFs were incubated with Ang II, a potent inducer of fibrosis, for 24 h. Irx2 and Irx3 expression was increased, while Irx4 expression was decreased in isolated CFs after Ang II treatment compared to control phosphate-buffered saline (PBS) treatment (Fig. 1A ). There were no differences in the other IRX members between the two groups. This finding was confirmed in human CFs, and we observed that IRX2 and IRX3 levels were also increased in Ang II-treated human CFs (Fig. 1B ). However, Ang II did not decrease IRX4 expression in human CFs. IRX2 was the IRX family member most consistently and significantly upregulated by Ang II stimulation. Consistent with these data, Irx2 mRNA expression were significantly increased in Ang II infusion-induced fibrotic hearts, which was indicated by increased mRNA levels of markers of fibrosis, including Col1 and α-Sma (Fig. 1C , Supplementary Fig. 1A ). Western blotting results suggested that IRX2 protein expression was increased in the hearts of mice following 12-week-Ang II infusion (Fig. 1D ). To enhance the clinical significance of our findings, we detected the expression of IRX2 in human heart samples from patients with DCM. The failing human hearts exhibited fibrosis, as reflected by increased TGF-β3 and α-SMA levels (Supplementary Fig. 1B ). As expected, IRX2 expression was significantly upregulated in the failing human hearts compared with control hearts (Fig. 1E ). In a recent report, Irx2 was also shown to be increased in a mouse model of DCM by RNA-seq [15] . IRX2 was mainly located in the nuclei of CFs (Supplementary Fig. 1C ). To identify the cellular source of upregulated IRX2 in fibrotic hearts, we fractionated endothelial cells, cardiomyocytes, and CFs from hearts treated with Ang II for 12 weeks to examine the expression pattern of Irx2 . Irx2 mRNA levels were much higher in CFs than in cardiomyocytes and endothelial cells (Fig. 1F ). Surprisingly, Ang II infusion had no significant effect on Irx2 mRNA expression in cardiomyocytes or endothelial cells but markedly increased Irx2 mRNA levels in CFs (Fig. 1F ). In agreement with this finding, immunofluorescence staining for IRX2, Collagen 1 (Col1, a marker for CFs), and cardiac Troponin T (cTnT, a marker for cardiomyocytes) revealed IRX2 expression in Col1-positive fibroblasts but not in cTnT-positive cardiomyocytes (Supplementary Fig. 1D ). Next, the IRX2 protein was evaluated in CFs isolated from the hearts of Ang II-infused mice. Compared with the CFs of saline-infused mice, the CFs isolated from mice treated with Ang II infusion showed significantly increased IRX2 protein expression (Fig. 1G ). We also found that periostin (POSTN) + /IRX2+ CFs were almost absent in saline or sham-treated hearts, but significantly increased after long-term pressure overload or Ang II infusion (Supplementary Fig. 1E-G ). Fig. 1: IRX2 expression was increased in fibrotic hearts. A Relative mRNA levels of 6 Irx family members in adult mouse cardiac fibroblasts (CFs) after angiotensin II (Ang II) treatment for 24 h ( n = 5). B Relative mRNA levels of 6 IRX family members in human CFs after Ang II treatment for 24 h ( n = 5). C Irx2 mRNA levels in the heart after Ang II infusion by an osmotic minipump ( n = 6). D Representative western blots and statistical analysis of IRX2 expression in the heart after Ang II infusion for 12 weeks ( n = 6). E Representative western blots and statistical analysis of IRX2 expression in heart samples obtained from patients with dilated cardiomyopathy (DCM) and control (Con) donors (Con, n = 6; DCM, n = 7). F Irx2 mRNA levels in endothelial cells (ECs), cardiomyocytes (CMs) and CFs isolated from hearts infused with Ang II for 12 weeks ( n = 6). G Representative western blots and quantification of IRX2 protein expression in CFs isolated from hearts infused with Ang II for 12 weeks ( n = 6). Data are shown as the mean ± SEM, and analysed using an unpaired two-tailed Student′s t test. For the analysis in ( C ), one-way ANOVA with Tamhane’s T2 test was conducted. Source data are provided as a Source Data file. Full size image IRX2 is a regulator of cardiac fibrosis in mice To investigate the effect of IRX2 on cardiac fibrosis, we performed 5 independent animal experiments to obtain the most conclusive evidence. First, mice with a conditional knockout allele of Irx2 ( Irx2 fl/fl ) were generated and crossed with tamoxifen-inducible Col1α2 -CreER mice ( Col1α2 -Cre) to obtain conditional fibroblast-specific Irx2 -deficient mice ( Irx2 cfKO) (Supplementary Fig. 2A ). Irx2 cfKO mice and control littermates were injected intraperitoneally with tamoxifen to induce the depletion of Irx2 in fibroblasts (Fig. 2A ). Irx2 cfKO mice were viable, fertile and phenotypically normal. After a 2-week washout period, mouse CFs freshly isolated from Irx2 cfKO mice demonstrated ∼ 61% IRX2 protein loss compared to CFs isolated from Irx2 fl/fl littermates (Fig. 2B ). However, the IRX2 protein expression in cardiomyocytes was unchanged (Supplementary Fig. 2B ). To further examine whether the expression of other Irx genes is affected in Irx2 -deficient CFs, we assessed the mRNA levels of other Irx genes in mouse CFs freshly isolated from Irx2 cfKO mice. No difference in the expression of Irx1 , Irx3 , Irx4 , Irx5 and Irx6 could be detected between CFs freshly isolated from Irx2 cfKO mice and CFs isolated from Irx2 fl/fl littermates (Supplementary Fig. 2C ). To determine the effects of IRX2 deficiency on cardiac fibrosis, Irx2 cfKO mice and littermate controls were subjected to 12 weeks of Ang II infusion. Upon Ang II infusion, the Irx2 cfKO mice exhibited a notable alleviation of cardiac enlargement compared with the Col1α2 -Cre and Irx2 fl/fl controls, as indicated by decreased heart weight-to-tibia length (HW/TL) ratio (Fig. 2C ). Irx2 cfKO mice exhibited reduced cardiac fibrosis after Ang II infusion compared with littermate controls, whereas no significant fibrosis was observed in the heart of Irx2 cfKO and littermate controls after saline infusion (Fig. 2D ). Ang II-induced cardiomyocyte hypertrophy was moderately attenuated in Irx2 cfKO mice compared with littermate controls (Fig. 2E ). Next, we detected the mRNA levels of two key fibrotic genes and found that Col1 and Col3 were upregulated in the heart of Col1α2 -Cre and Irx2 fl/fl littermate controls by Ang II infusion and that this induction was largely attenuated in Irx2 cfKO mice (Fig. 2F ). Immunoblotting results then confirmed that the Ang II infusion-induced protein levels of α-SMA and connective tissue growth factor (CTGF) were blocked by fibroblast-specific depletion of Irx2 in mice (Supplementary Fig. 3A ). The transcriptional levels of hypertrophic markers, including Anp , Bnp and β-Mhc , were significantly suppressed in heart samples from Irx2 cfKO mice compared with heart samples from littermate controls (Supplementary Fig. 3B ). Furthermore, echocardiographic assessment of cardiac function indicated that fibroblast-specific Irx2 depletion attenuated Ang II-induced cardiac dysfunction, as evidenced by an elevated ejection fraction (EF) and a decreased left ventricular end-diastolic dimension (LVIDd) and interventricular septal thickness at diastole (IVSd) (Fig. 2G , Supplementary Fig. 3C ). Ang II infusion induced an increase in systolic blood pressure in Irx2 cfKO mice and littermate controls; however, there was no significant difference in systolic blood pressure among all three groups (Supplementary Fig. 3D ). The heart rate was unchanged in Irx2 cfKO mice and littermate controls after Ang II infusion for (Supplementary Fig. 3E ). Fig. 2: Conditional fibroblast-specific Irx2 -deficient mice exhibited attenuated fibrotic remodelling in response to angiotensin II (Ang II) infusion. A Conditional fibroblast-specific Irx2 -deficient mice ( Irx2 cfKO) were bred by crossing mice with a conditional knockout allele of Irx2 ( Irx2 fl/fl ) with Col1α2 -Cre mice. Irx2 cfKO mice and littermate controls were subjected to Ang II infusion for 12 weeks. B Representative western blots and statistical analysis of IRX2 protein expression in CFs isolated from Irx2 cfKO mice and littermate controls ( n = 5). C – E Irx2 cfKO mice exhibited an attenuated heart weight-to-tibia length (HW/TL) ratio ( n = 10 mice, Col1α2 -Cre+Saline; n = 12 mice, Irx2 fl/fl +Saline; n = 12 mice, Irx2 cfKO+Saline; n = 12 mice, Col1α2 -Cre+Ang II; n = 11 mice, Irx2 fl/fl +Ang II; n = 12 mice, Irx2 cfKO+Ang II) ( C ), a reduced fibrosis area ( n = 5) ( D ), and a decreased cell area of cardiomyocytes ( n = 5) ( E ) after Ang II infusion. F Relative mRNA levels of Col1 and Col3 in hearts from Irx2 cfKO mice and littermate controls after Ang II infusion ( n = 6). G Cardiac function ( n = 6) was improved in Ang II-infused Irx2 cfKO mice. Data are shown as the mean ± SEM, and analysed using one-way ANOVA followed by Tukey post hoc test ( E and G ) or Tamhane’s T2 test ( C , D and F ). For the analysis in ( B ), an unpaired two-tailed Student′s t test was conducted. Source data are provided as a Source Data file. Full size image Second, we generated injury-inducible myofibroblast-specific Irx2 -knockout mice ( Irx2 mfKO). In the healthy adult heart, periostin expression is negligible [16] , [17] . Upon injury, periostin expression is robustly increased and specifically marks activated myofibroblasts in the fibrotic heart [16] , [17] . Periostin is not present in resident CFs, cardiomyocytes, endothelial cells, vascular smooth muscle cells or inflammatory cells [5] , [16] , [18] and thus can be used for the specific manipulation of activated myofibroblasts. To generate injury-inducible Irx2 mfKO mice, Irx2 fl/fl mice were bred with Postn -Cre mice. Irx2 mfKO mice were also viable, fertile and phenotypically normal. Irx2 mfKO mice were subjected to 12 weeks of Ang II infusion (Fig. 3A ). To investigate the extent of Postn -Cre-mediated Irx2 deletion, we isolated CFs from Ang II-infused Irx2 mfKO mice and found that the IRX2 protein level was reduced by ∼ 73% in these mice compared to littermate controls (Fig. 3B ). However, the Irx2 mRNA level in cardiomyocytes was unchanged (Supplementary Fig. 4A ). Consistent with the findings for Irx2 cfKO mice, Irx2 mfKO mice exhibited alleviated fibrotic remodelling upon Ang II infusion, as indicated by reductions in the HW/TL ratio, fibrosis area, cell area of cardiomyocytes and levels of fibrotic markers ( Col1 and Col3 mRNA levels), compared with littermate controls (Fig. 3C-F ). The increased protein expression of α-SMA and CTGF induced by Ang II infusion was also suppressed by myofibroblast-specific depletion of Irx2 in mice (Supplementary Fig. 4B ). We also found that myofibroblast-specific depletion of Irx2 decreased the number of POSTN + /IRX2+ cells in response to Ang II infusion (Supplementary Fig. 4C ). Further detection of the mRNA levels of hypertrophic markers revealed that myofibroblast-specific depletion of Irx2 inhibited the pathological elevations in these hypertrophic markers in Ang II-treated mice (Supplementary Fig. 4D ). Compared with Postn -Cre and Irx2 fl/fl control mice, Irx2 mfKO mice showed improved cardiac function after Ang II infusion, as indicated by an elevated EF and a reduced LVIDd (Fig. 3G, H ). Fig. 3: Conditional myofibroblast-specific Irx2 depletion attenuated angiotensin II (Ang II) or pressure overload-induced cardiac fibrosis in mice. A Conditional myofibroblast-specific Irx2 -deficient mice ( Irx2 mfKO) were bred by crossing mice with a conditional knockout allele of Irx2 ( Irx2 fl/fl ) with Postn -Cre mice. Irx2 mfKO mice and littermate controls were subjected to Ang II infusion for 12 weeks. B Representative western blots and statistical analysis of IRX2 protein expression in CFs isolated from Irx2 mfKO mice and littermate controls after Ang II infusion for 12 weeks ( n = 5). C Heart weight-to-tibia length (HW/TL) ratio ( n = 10 mice, Postn -Cre+Saline; n = 11 mice, Irx2 fl/fl +Saline; n = 11 mice, Irx2 mfKO+Saline; n = 10 mice, Postn -Cre+Ang II; n = 12 mice, Irx2 fl/fl +Ang II; n = 12 mice, Irx2 mfKO+Ang II). D Cardiac fibrosis was determined by picrosirius red staining for Irx2 mfKO mice after Ang II infusion for 12 weeks ( n = 5). E The cell area of cardiomyocytes was determined with wheat germ agglutinin (WGA) staining for Irx2 mfKO and littermate controls after Ang II infusion for 12 weeks ( n = 5). F The relative mRNA levels of Col1 and Col3 were detected in hearts from Irx2 mfKO mice and control mice ( n = 6). G , H The ejection fraction (EF) ( G ) and left ventricular end-diastolic dimension (LVIDd) ( H ) were detected in these groups ( n = 6). I Irx2 mfKO mice and littermate controls were subjected to transverse aortic constriction (TAC) surgery for 6 weeks. J HW/TL ratio ( n = 10 mice, Postn -Cre+Sham; n = 11 mice, Irx2 fl/fl +Sham; n = 11 mice, Irx2 mfKO+Sham; n = 10 mice, Postn -Cre+TAC; n = 12 mice, Irx2 fl/fl + TAC; n = 12 mice, Irx2 mfKO+TAC). K Histological staining showing cardiac fibrosis after TAC surgery in Irx2 mfKO mice ( n = 5). L Cell area of cardiomyocytes determined with WGA staining after TAC surgery ( n = 5). M , N EF ( M ) and LVIDd ( N ) detected in these groups ( n = 8).The data were compared by one-way ANOVA. Data are shown as the mean ± SEM, and analysed using one-way ANOVA followed by Tukey post hoc test ( D – H and L – N ) or Tamhane’s T2 test ( C , and J – K ). For the analysis in ( B ), an unpaired two-tailed Student′s t test was conducted. Source data are provided as a Source Data file. Full size image Third, in addition to Ang II infusion, pressure overload is another well-studied mouse model of cardiac fibrosis [19] . To exclude the possibility that the pro-fibrotic effect of IRX2 is specific to Ang II-induced cardiac fibrosis, we next investigated whether myofibroblast-specific depletion of Irx2 could attenuate pressure overload-induced fibrotic remodelling in vivo (Fig. 3I ). Mice subjected to pressure overload developed cardiac hypertrophy and fibrosis, as indicated by increases in the HW/TL ratio, cardiomyocyte cell area and fibrosis area (Fig. 3J-L ). Irx2 mfKO mice exhibited moderate declines in the HW/TL ratio and cardiomyocyte cell area but a robust decline in the fibrosis area in response to pressure overload (Fig. 3J-L ). The increased EF and decreased LVIDd indicated attenuated cardiac dysfunction in Irx2 mfKO mice compared with control littermates in response to pressure overload (Fig. 3M, N ). Fourth, we generated cardiomyocyte-specific Irx2 -knockout mice ( Irx2 cmKO) to exclude the effect of cardiomyocyte-derived IRX2 on fibrotic remodelling (Supplementary Fig. 5A ). Irx2 cmKO mice were generated by crossing Irx2 fl/fl mice with α-Mhc -Cre mice. Mouse cardiomyocytes freshly isolated from Irx2 cmKO demonstrated ∼ 55% IRX2 protein loss compared to cardiomyocytes isolated from IRX2 fl/fl littermates (Supplementary Fig. 5A ). However, the Irx2 mRNA in CFs was unchanged (Supplementary Fig. 5B ). We found that Ang II infusion for 12 weeks induced an increase in the HW/TL ratio, cell area of cardiomyocytes and fibrosis area; however, these pathological alterations were not attenuated by cardiomyocyte-specific depletion of Irx2 (Supplementary Fig. 5C-F ). Cardiomyocyte-specific depletion of Irx2 did not attenuate Ang II-induced cardiac dysfunction, as indicated by the similar EF among the three Ang II-infused groups (Supplementary Fig. 5G ). Finally, we pursued a gain-of-function approach. We further investigated whether overexpressing Irx2 in myofibroblasts promoted Ang II-induced cardiac fibrosis in vivo by generating myofibroblast-specific Irx2 transgenic mice ( Irx2 mfTg). To achieve this, conditional transgenic founder mice expressing the Irx2 gene ( Irx2 Tg fl/fl ) were bred with Postn -Cre mice. This experimental design sketch was showed in Fig. 4A . To prevent potential contamination caused by transgenic leakiness, we evaluated IRX2 protein expression in several organs of Irx2 mfTg mice and Irx2 Tg fl/fl littermates after Ang II infusion. In response to Ang II infusion, IRX2 was increased only in the heart of Irx2 mfTg mice (Supplementary Fig. 6A ), confirming the integrity and specificity of this overexpression system. We also found that IRX2 protein expression was significantly increased in myofibroblasts freshly isolated from Ang II-infused Irx2 mfTg mice compared with myofibroblasts isolated from Irx2 Tg fl/fl littermates (Fig. 4B ). However, IRX2 protein expression in cardiomyocytes was unchanged (Supplementary Fig. 6B ). As expected, overexpression of Irx2 in myofibroblasts moderately increased the HW/TL ratio and cell area of cardiomyocytes but robustly increased the fibrosis area in Ang II-infused mice (Fig. 4C-E ). Accordingly, the mRNA levels of Col1 and Col3 , as well as the protein expression of α-SMA, were higher in Irx2 mfTg mice than in control littermates upon Ang II infusion (Fig. 4F , Supplementary Fig. 6C-D ). We also found that myofibroblast-specific overexpression of Irx2 increased the number of POSTN + /IRX2+ myofibroblasts in response to Ang II infusion (Supplementary Fig. 6E ). Ang II infusion for 4 weeks could induce cardiac hypertrophy and fibrosis without altering the EF [20] , [21] . Consistent with these reports, mice infused with Ang II for 4 weeks exhibited an unaltered EF and LVIDd. Mice with conditional myofibroblast-specific overexpression of Irx2 had a decreased EF and an increased LVIDd after 4 weeks of Ang II infusion (Fig. 4G, H ). Taken together, these results suggested that CF-derived IRX2, not cardiomyocytes, contributed to Ang II-induced fibrotic remodelling in mice. Fig. 4: Conditional myofibroblast-specific Irx2 overexpression promoted angiotensin II (Ang II)-induced fibrotic remodelling in mice. A Conditional myofibroblast-specific Irx2 -overexpressing mice ( Irx2 mfTg) were bred by crossing conditional transgenic mice expressing the Irx2 gene ( Irx2 Tg fl/fl ) with Postn -Cre mice. Irx2 mfTg mice and their littermate controls were subjected to Ang II infusion for 4 weeks. B Representative western blots and statistical analysis of IRX2 protein expression in CFs isolated from Irx2 mfTg mice and littermate controls after Ang II infusion for 4 weeks ( n = 5). C Heart weight to tibia length (HW/TL) ratio ( n = 12 mice for all six groups). D Cardiac fibrosis was determined by picrosirius red staining in Irx2 mfTg mice after Ang II infusion ( n = 5). E Cell area of cardiomyocytes was determined with wheat germ agglutinin (WGA) staining in Irx2 mfTg and littermate controls after Ang II infusion ( n = 5). F Relative mRNA levels of Col1 and Col3 were detected in the hearts of Irx2 mfTg mice and their controls ( n = 6). G , H Ejection fraction (EF) ( G ) and left ventricular end-diastolic dimension (LVIDd) ( H ) were detected in these groups ( n = 6). The data were compared by one-way ANOVA. Data are shown as the mean ± SEM, and analysed using one-way ANOVA followed by Tukey post hoc test ( C – D and G – H ) or Tamhane’s T2 test ( E – F ). For the analysis in ( B ), an unpaired two-tailed Student′s t test was conducted. Source data are provided as a Source Data file. Full size image IRX2 is required for cardiac fibroblast-to-myofibroblast conversion Next, we investigated the direct effects of IRX2 deletion on the phenotype of CFs. Adult CFs were isolated from Irx2 fl/fl mouse hearts, and Irx2 depletion was achieved by adenovirus-mediated Cre expression. Cre infection led to an ∼ 87% reduction in IRX2 protein expression in vitro (Fig. 5A ). Irx2 depletion significantly decreased α-Sma expression in the presence of Ang II (Fig. 5B ). Immunofluorescence analysis also revealed that the Irx2 depletion mediated by Cre expression decreased the α-SMA fluorescence intensity in Ang II-treated CFs (Fig. 5C ). We also found that conditioned medium from CFs isolated from Irx2 cfKO mice significantly attenuated Ang II-induced cardiomyocyte hypertrophy in vitro (Supplementary Fig. 7A ). In addition to the Cre-mediated deletion approach, we used an shRNA-mediated interference approach. Two small hairpin RNAs (shRNAs) targeting Irx2 (sh Irx2 #1 and #2) significantly decreased IRX2 protein expression in wild-type (WT) mouse CFs (Supplementary Fig. 7B ). This shRNA-mediated knockdown of Irx2 significantly suppressed the upregulation of α-SMA+ cells in response to Ang II treatment (Fig. 5D ). In addition, two shRNAs against Irx2 (#1 and #2) decreased Ang II-induced Col1 production in CFs (Fig. 5E ). Next, we evaluated whether Irx2 deficiency affects CF proliferation. IRX2 did not affect CF proliferation upon 5% fetal bovine serum (FBS) or Ang II administration (Supplementary Fig. 7C, D ). In line with the above findings, we found that Irx2 overexpression aggravated the Ang II-induced transdifferentiation of fibroblasts into myofibroblasts, as suggested by the increased α-SMA expression in CFs isolated from WT mice (Fig. 5F , Supplementary Fig. 7E ). A gain-of-function experiment was also performed with human CFs. Consistent with the findings for mouse CFs, IRX2 overexpression promoted the Ang II-induced transdifferentiation of fibroblasts into myofibroblasts, which was reflected by increased mRNA levels of Col1 , α-Sma and Postn (Supplementary Fig. 7F, G ). Next, we performed gene profiling of Irx2 -overexpressing mouse CFs and control CFs after Ang II administration using RNA-seq assays. Under the conditions of fold change >1.1 and adjusted P value (padj) <0.01, we found that 2431 genes were upregulated and 2199 genes were downregulated in Irx2 -overexpressing CFs compared with control CFs after Ang II treatment (Fig. 5G ). The heatmap results revealed that the expression of fibrosis-related genes was significantly upregulated in Irx2 -overexpressing CFs compared with control CFs (Fig. 5H ). Some of these upregulated genes were key mediators of the Ang II-induced fibrotic response, including Tgf-β3, Pdgf-a, Pdgf-b, Smad3, Col1a1, Tipm3 and several Fgf family genes (Fig. 5H , Supplementary Table 2 ). 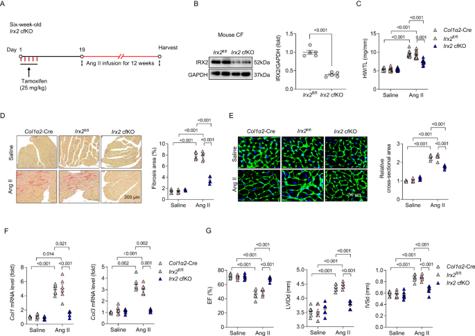Fig. 2: Conditional fibroblast-specificIrx2-deficient mice exhibited attenuated fibrotic remodelling in response to angiotensin II (Ang II) infusion. AConditional fibroblast-specificIrx2-deficient mice (Irx2cfKO) were bred by crossing mice with a conditional knockout allele ofIrx2(Irx2fl/fl) withCol1α2-Cre mice.Irx2cfKO mice and littermate controls were subjected to Ang II infusion for 12 weeks.BRepresentative western blots and statistical analysis of IRX2 protein expression in CFs isolated fromIrx2cfKO mice and littermate controls (n= 5).C–EIrx2cfKO mice exhibited an attenuated heart weight-to-tibia length (HW/TL) ratio (n= 10 mice,Col1α2-Cre+Saline;n= 12 mice,Irx2fl/fl+Saline;n= 12 mice,Irx2cfKO+Saline;n= 12 mice,Col1α2-Cre+Ang II;n= 11 mice,Irx2fl/fl+Ang II;n= 12 mice,Irx2cfKO+Ang II) (C), a reduced fibrosis area (n= 5) (D), and a decreased cell area of cardiomyocytes (n= 5) (E) after Ang II infusion.FRelative mRNA levels ofCol1andCol3in hearts fromIrx2cfKO mice and littermate controls after Ang II infusion (n= 6).GCardiac function (n= 6) was improved in Ang II-infusedIrx2cfKO mice. Data are shown as the mean ± SEM, and analysed using one-way ANOVA followed by Tukey post hoc test (EandG) or Tamhane’s T2 test (C,DandF). For the analysis in (B), an unpaired two-tailed Student′sttest was conducted. Source data are provided as a Source Data file. Gene Ontology (GO) term analysis of differentially expressed genes (DEGs) revealed that several signalling pathways were closely related to fibrotic remodelling, specifically cadherin binding, cell adhesion molecule binding, cell–cell junction, focal adhesion, adherens junction, anchoring junction and cell growth (Supplementary Fig. 8A ). Reactome term analysis also identified several pro-fibrotic classes, such as assembly of collagen fibrils, extracellular matrix organization, TGF-β receptor signalling, PDGF signalling pathway, vascular endothelial growth factor (VEGF) signalling pathway, ephrin B-mediated forward signalling, Wnt ligand biogenesis and trafficking, and cell–cell communication (Supplementary Fig. 8B ). Fig. 5: IRX2 is essential for fibroblast to myofibroblast transformation. A Adult cardiac fibroblasts (CFs) were isolated from Irx2 fl/fl mice and infected with an adenoviral vector carrying Cre to deplete Irx2 . After 24 h of transfection, IRX2 protein expression was detected in CFs ( n = 5). B Relative mRNA level of α-Sma in Irx2 -depleted adult mouse CFs ( n = 5). C Representative images and quantification of α-SMA (green) in Cre-infected Irx2 fl/fl CFs in response to Ang II incubation for 24 h. Nuclei are stained with DAPI (blue). ( n = 5, for each group, 50-60 fields were counted). D CFs were isolated from wild-type mice and then transfected with shRNAs targeting Irx2 . After 24 h of transfection, the cells were subjected to Ang II treatment for 24 h to induce a fibrotic phenotype. After that, the cells were harvested for the detection of α-SMA with western blotting ( n = 4). E Relative mRNA level of Col1 in IRX2-deficient CFs after Ang II incubation for 24 h ( n = 4). F CFs were isolated from wild-type mice and then overexpressed Irx2 with an adenovirus vector, after which they were subjected to Ang II treatment for 24 h. The relative mRNA level of α-Sma was detected to reflect fibroblast to myofibroblast transformation ( n = 5). G CFs were isolated from wild-type mice and then overexpressed Irx2 with an adenovirus vector, after which they were subjected to Ang II treatment for 24 h. Total RNA was extracted, and RNA sequencing was performed. Volcano plots indicating the differentially expressed genes (DEGs) in Irx2 -overexpressing CFs relative to controls after Ang II administration for 24 h. H Heatmap of several differentially expressed genes in Irx2 -overexpressing CFs relative to controls after Ang II infusion. Data are shown as the mean ± SEM, and analysed using one-way ANOVA followed by Tukey post hoc test ( B and D – F ) or Tamhane’s T2 test ( C ). For the analysis in ( A ), an unpaired two-tailed Student′s t test was conducted. Source data are provided as a Source Data file. Full size image EGR1 was identified as a direct downstream target gene of IRX2 To explore how IRX2 regulates fibrotic remodelling, we identified the downstream targets of IRX2 by chromatin immunoprecipitation-sequencing (ChIP-seq) with two anti-IRX2 antibodies (IRX2-1B7 and IRX2-1C1). Human CFs were infected with an adenovirus carrying IRX2 and then subjected to Ang II stimulation. Overexpression of IRX2 was confirmed by western blotting (Supplementary Fig. 7F ). A similar spatial distribution of IRX2 peaks was identified for each of the two IRX2 antibodies (Fig. 6A ). ChIP-seq using IRX2-1B7 revealed that the peaks distributed in the promoter transcription site comprised 25.59% of the total peaks, while ChIP-seq using IRX2-1C1 revealed that the peaks distributed in the promoter site comprised 31.41% of the total peaks (Supplementary Fig. 9A, B ). Then, a bioinformatic intersection analysis between the upregulated DEGs identified by RNA-sequencing (RNA-seq) and enriched genes revealed to be within the promoter transcription site by ChIP-seq was performed, and 70 genes were identified (Fig. 6B , Supplementary Table 3 ). 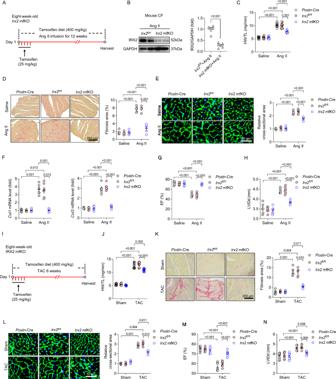Fig. 3: Conditional myofibroblast-specificIrx2depletion attenuated angiotensin II (Ang II) or pressure overload-induced cardiac fibrosis in mice. AConditional myofibroblast-specificIrx2-deficient mice (Irx2mfKO) were bred by crossing mice with a conditional knockout allele ofIrx2(Irx2fl/fl) withPostn-Cre mice.Irx2mfKO mice and littermate controls were subjected to Ang II infusion for 12 weeks.BRepresentative western blots and statistical analysis of IRX2 protein expression in CFs isolated fromIrx2mfKO mice and littermate controls after Ang II infusion for 12 weeks (n= 5).CHeart weight-to-tibia length (HW/TL) ratio (n= 10 mice,Postn-Cre+Saline;n= 11 mice,Irx2fl/fl+Saline;n= 11 mice,Irx2mfKO+Saline;n= 10 mice,Postn-Cre+Ang II;n= 12 mice,Irx2fl/fl+Ang II;n= 12 mice,Irx2mfKO+Ang II).DCardiac fibrosis was determined by picrosirius red staining forIrx2mfKO mice after Ang II infusion for 12 weeks (n= 5).EThe cell area of cardiomyocytes was determined with wheat germ agglutinin (WGA) staining forIrx2mfKO and littermate controls after Ang II infusion for 12 weeks (n= 5).FThe relative mRNA levels ofCol1andCol3were detected in hearts fromIrx2mfKO mice and control mice (n= 6).G,HThe ejection fraction (EF) (G) and left ventricular end-diastolic dimension (LVIDd) (H) were detected in these groups (n= 6).IIrx2mfKO mice and littermate controls were subjected to transverse aortic constriction (TAC) surgery for 6 weeks.JHW/TL ratio (n= 10 mice,Postn-Cre+Sham;n= 11 mice,Irx2fl/fl+Sham;n= 11 mice,Irx2mfKO+Sham;n= 10 mice,Postn-Cre+TAC;n= 12 mice,Irx2fl/fl+ TAC;n= 12 mice,Irx2mfKO+TAC).KHistological staining showing cardiac fibrosis after TAC surgery inIrx2mfKO mice (n= 5).LCell area of cardiomyocytes determined with WGA staining after TAC surgery (n= 5).M,NEF (M) and LVIDd (N) detected in these groups (n= 8).The data were compared by one-way ANOVA. Data are shown as the mean ± SEM, and analysed using one-way ANOVA followed by Tukey post hoc test (D–HandL–N) or Tamhane’s T2 test (C, andJ–K). For the analysis in (B), an unpaired two-tailed Student′sttest was conducted. Source data are provided as a Source Data file. We selected the upregulated DEGs in the RNA-seq data because IRX2 acted as a transcriptional activator after activation by mitogen-activated protein kinases [13] . Next, we excluded genes with low abundance in the heart and molecules that have never been related to cardiovascular diseases. After that, the number of IRX2-enriched genes was narrowed to 10. The genes were Gadd45β, Paxillin, Vegfα, Egr1, Nectin2, Serpine2, Klf10, Dusp5, Mapkapk3 and Col6a2 . Five of them ( Gadd45β , Gadd45β , Nectin2 , Klf10 and Dusp5 ) have been reported to protect against fibrotic remodelling [22] , [23] , [24] , [25] , [26] ; thus, they were not the molecules responsible for the pro-fibrotic effects of IRX2. We focused our interest on EGR1 for the reason that EGR1 is a key transcription factor in fibrotic diseases [27] . Increased EGR1 expression were observed in several animal models of fibrosis and human fibrotic diseases [27] . Egr1 -deficient mice were protected from bleomycin-induced skin and lung fibrosis [28] . More importantly, several EGR1-regulated signalling pathways have been revealed by Reactome term analysis of RNA-seq data, such as assembly of collagen fibrils, extracellular matrix organization, TGF-β receptor signalling, PDGF signalling pathway, VEGF signalling pathway and Wnt signalling pathway [27] , [29] . IRX2 acted as a transcriptional factor by specifically binding to the ACAnnTGT motif of target genes [30] , [31] . When searching this motif (ACAnnTGT) among the ChIP-seq peak distributed in the promoter site of Egr1 , we found that there was two IRX2 binding sites (Fig. 6C ). Next, we performed a luciferase assay with mouse CFs. Irx2 overexpression dramatically increased luciferase activity in CFs in a dose-dependent manner, suggesting that IRX2 directly stimulated the transcription of Egr1 (Fig. 6D ). More important, after these IRX2 binding sites were mutated, IRX2-mediated upregulation of luciferase activity was abrogated (Fig. 6E ). To corroborate this finding, ChIP-PCR was performed with Ang II-treated mouse CFs, and the results showed enrichment of the Egr1 promoter region in the IRX2 precipitate (Fig. 6F ). These results suggested that EGR1 was a direct transcriptional target of IRX2. Consistent with these in vitro findings, Egr1 mRNA and protein expression were decreased in CFs isolated from Irx2 cfKO mice in comparison with those isolated from Col1α2 -Cre and Irx2 fl/fl littermate controls after Ang II infusion (Fig. 6G-H ). Using a Cre-mediated deletion approach, we also found that Irx2 deficiency inhibited the pathological elevation in EGR1 in Ang II-treated Irx2 fl/fl CFs (Fig. 6I ). Conversely, CFs isolated from Ang II-infused Irx2 mfTg mice exhibited significantly elevated expression of EGR1 compared with CFs isolated from Ang II-infused Postn -Cre and Irx2 Tg fl/fl mice (Fig. 6J, K ). Using human CFs, we also confirmed that IRX2 overexpression increased EGR1 mRNA expression in Ang II-treated CFs (Fig. 6L ). Fig. 6: EGR1 was identified as a direct downstream target gene of IRX2 in cardiac fibroblasts that regulates the angiotensin II (Ang II)-induced fibrotic response. A CFs were infected with an adenovirus carrying IRX2 and then subjected to Ang II stimulation for 24 h. ChIP-seq was performed with two anti-IRX2 antibodies (IRX2-1B7 and IRX2-1C1). Similar spatial distributions of IRX2 peaks were identified by the two anti-IRX2 antibodies. B IRX2-regulated genes identified in the ChIP-seq data (bottom) were overlaid with upregulated differentially expressed genes revealed by RNA-seq (top). With this strategy, 70 genes were identified. C Two IRX2 binding sites were identified in the ChIP-seq peak distributed in the promoter site of Egr1 . D The Egr1 promoter was stimulated by IRX2 overexpression. Egr1 promoter activity was measured by a luciferase assay upon Irx2 overexpression in CFs isolated from wild-type mice ( n = 5 for each group). E The mutant (Mut) promoters (pro) deleting IRX2 binding sites cannot be stimulated by Irx2 overexpression ( n = 5 for each group). F Independent ChIP-PCR was performed with Irx2 -overexpressing CFs to verify IRX2 binding to the promoter of Egr1 ( n = 5). G – H Egr1 mRNA and EGR1 protein expression in CFs isolated from Irx2 cfKO mice and littermate controls with or without Ang II infusion for 12 weeks ( n = 6). I Egr1 mRNA levels were detected in CFs with Irx2 deficiency caused by Cre expression ( n = 5). J – K Egr1 mRNA and EGR1 protein expression in CFs isolated from Irx2 mfTg mice and littermate controls with or without Ang II infusion for 4 weeks ( n = 6). L Egr1 mRNA level in Irx2 -overexpressing human CFs after Ang II treatment for 24 h ( n = 6). Data are shown as the mean ± SEM, and analysed using one-way ANOVA followed by Tukey post hoc test ( H , I and K ) or Tamhane’s T2 test ( D – G , J and L ). Source data are provided as a Source Data file. Full size image IRX2 regulated cardiac fibrosis via an EGR1-dependent mechanism To determine the requirement for EGR1 in the IRX2-mediated fibrotic response, CFs were isolated from Irx2 Tg fl/fl mice and infected with an adenovirus carrying Cre to overexpress IRX2. After that, EGR1 expression was knocked down. Egr1 deficiency abolished the IRX2-promoted transdifferentiation of fibroblasts into myofibroblasts in vitro (Supplementary Fig. 10A , Fig. 7A ). Ang II-induced collagen accumulation, as reflected by Col1 and Col3 mRNA levels, was enhanced by the overexpression of Irx2 , and this effect of Irx2 was blocked by Egr1 knockdown (Fig. 7B, C ). To further confirm the role of EGR1 in the IRX2-mediated fibrotic response, we isolated CFs from Egr1 global knockout mice. These cells were then infected with an adenovirus carrying Irx2 . EGR1 protein expression was absent in CFs isolated from Egr1 -deficient mice (Supplementary Fig. 10B ). The results demonstrated that IRX2 did not enhance the Ang II-induced transdifferentiation of fibroblasts into myofibroblasts in Egr1 -deficient CFs (Fig. 7D , Supplementary Fig. 10C ). Consistent with the above findings, after these IRX2 binding sites were mutated, IRX2-mediated effect was abrogated, as reflected by α-Sma mRNA level (Fig. 7E ). To establish a causative relationship between EGR1 and fibrotic remodelling, we performed an Egr1 gain-of-function experiment with isolated CFs. Egr1 overexpression in CFs resulted in spontaneous myofibroblast transdifferentiation (Supplementary Fig. 10D ). EGR1 could bind to the promoters of Tgf-β3 , Pdgf-a , Pdgf-b , Col1α2 , Pai-1 and Timp3 and increase the expression of these downstream genes [27] . We also found that Egr1 overexpression significantly increased the mRNA levels of Tgf-β3 , Pdgf-a , Pdgf-b , Col1α2 , Pai-1 and Timp3 (Supplementary Fig. 10E ). As expected, Irx2 depletion significantly decreased the Ang II-induced pathological increases in TGF-β3, PDGF-A, PDGF-B, and PAI-1 in CFs (Fig. 7F ). Conversely, the Ang II-induced pathological elevations in Tgf-β3 , Pdgf-a , Pdgf-b , and Pai-1 were enhanced by overexpression of Irx2 in mouse CFs, and these effects could be blocked by Egr1 knockdown (Fig. 7G ). TGF-β3, PDGF and PAI-1 are known to activate Smad-3, which is likely to be a key driving factor in fibrosis [7] , [32] . Next, we determined the phosphorylation of Smad3 in isolated CFs. As hypothesized, Irx2 deficiency led to a significant reduction in the phosphorylation of Smad3 in CFs isolated from Irx2 cfKO or Irx2 mfKO mice after Ang II infusion (Fig. 7H, I ). Fig. 7: EGR1 was responsible for the IRX2-promoted fibrotic response in angiotensin II (Ang II)-treated cardiac fibroblasts. A – C Cardiac fibroblasts (CFs) were isolated from Irx2 Tg fl/fl mice and infected with an adenovirus carrying Cre to overexpress Irx2 . After that, Egr1 expression was knocked down, and the CFs were subjected to Ang II treatment for 24 h. After that, the cells were harvested to detect the mRNA levels of α-Sma ( A ), Col1 ( B ) and Col3 ( C ) ( n = 5). D Representative images of α-SMA (green) in CFs isolated from Egr1 -knockout mice after Ang II treatment for 24 h. Nuclei were stained with DAPI (blue) ( n = 5, for each experiment, 50-60 fields were counted). E Relative mRNA levels of α-Sma in the indicated groups ( n = 5). F Relative mRNA levels of fibrosis-related genes in CFs isolated from Irx2 cfKO mice and littermate controls with or without Ang II infusion for 12 weeks ( n = 5). G CFs were isolated from Irx2 Tg fl/fl mice and infected with an adenovirus carrying Cre to overexpress Irx2 . After that, Egr1 expression was knocked down, and the CFs were subjected to Ang II treatment for 24 h. After that, the cells were harvested to detect the mRNA levels of fibrosis-related genes ( n = 5). H , I Western blot analysis was performed to analyse the phosphorylation of Smad3 in CFs isolated from Irx2 cfKO or Irx2 mfKO mice and corresponding littermate controls with or without Ang II infusion for 12 weeks ( n = 6). Data are shown as the mean ± SEM, and analysed using one-way ANOVA followed by Tukey post hoc test ( A , C , E and G ) or Tamhane’s T2 test ( B , F , H and I ). Source data are provided as a Source Data file. Full size image Genetic depletion of Egr1 attenuated Ang II-induced cardiac fibrosis and improved cardiac function in Irx2 mfTg mice Finally, we confirmed the mechanisms underlying the observed pathological phenotype in Irx2 mfTg mice, with our hypothesis being that upregulation of EGR1 and its downstream pro-fibrotic genes in IRX2 mfTg mice is the cause, rather than a consequence, of this pathological fibrotic phenotype. To verify this, we evaluated whether genetic depletion of Egr1 could rescue the observed pathological phenotype in IRX2 mfTg mice after Ang II infusion. IRX2 mfTg mice or IRX2 Tg fl/fl littermates were bred with Egr1 -deficient mice. To our surprise, genetic depletion of Egr1 largely abolished the pathological phenotype caused by conditional myofibroblast-specific overexpression of IRX2, as evidenced by decreases in the HW/TL ratio, cardiomyocyte cell area and fibrosis area (Fig. 8A-D ). Genetic depletion of Egr1 blunted the Ang II-induced increase in fibrosis markers more in the heart of IRX2 mfTg mice than in IRX2 Tg fl/fl mice (Supplementary Fig. 11A-E ). Genetic depletion of Egr1 also partly restored ventricular function and chamber dimensions (Fig. 8E, F ). Together, these findings provide strong evidence that EGR1 upregulation is responsible for the pathological phenotype caused by conditional myofibroblast-specific overexpression of IRX2 in mice. Fig. 8: Genetic depletion of Egr1 attenuated fibrotic remodelling in mice with conditional myofibroblast-specific Irx2 overexpression after angiotensin II (Ang II) infusion. Conditional myofibroblast-specific Irx2 -overexpressing mice ( Irx2 mfTg) were bred with Egr1 global knockout mice or wild type (WT). The resulting mouse line and littermate controls were subjected to Ang II infusion for 4 weeks. A Heart weight-to-tibia length (HW/TL) ratio ( n = 10 mice, Irx2 Tg fl/fl + WT+Ang II; n = 10 mice, Irx2 Tg fl/fl + Egr1 KO+Ang II; n = 11 mice, Irx2 mfTg+WT+Ang II; n = 11 mice, Irx2 mfTg+ Egr1 KO+Ang II). B Histological staining showed cardiomyocyte enlargement and cardiac fibrosis after Ang II infusion ( n = 5). C Cardiac fibrosis was determined by picrosirius red staining after Ang II infusion ( n = 5). D The cell area of cardiomyocytes was determined with wheat germ agglutinin (WGA) staining after Ang II infusion ( n = 5). E , F The ejection fraction (EF) ( E ) and left ventricular end-diastolic dimension (LVIDd) ( F ) were detected in these groups ( n = 6). Data are shown as the mean ± SEM, and analyzed using one-way ANOVA followed by Tukey post hoc test ( A , C , and D ). For the analysis in ( E , F ), repeated measures ANOVA was conducted. Source data are provided as a Source Data file. Full size image Currently, although several pharmacological agents have been shown to be effective in heart failure, clinical strategies specifically for the treatment of cardiac fibrosis are not available. Identifying the molecular mechanisms of cardiac fibrosis will pave the way for developing new strategies for the treatment of cardiac remodelling. Herein, we report a detrimental role for IRX2 in the development of fibrosis. Specifically, fibroblast-specific Irx2 deletion attenuated two different heart fibrotic diseases and improved cardiac function. Myofibroblast-specific Irx2 gain of function promoted progressive cardiac fibrosis induced by Ang II and accelerated the deterioration of cardiac function in mice. Mechanistic studies demonstrated that IRX2 could directly bind to the promoter region of the Egr1 gene and subsequently activate downstream pro-fibrotic genes. Our study highlighted the possibility of developing therapeutic strategies targeting IRX2 to attenuate cardiac fibrosis. Irrespective of the initial cause, injury evoked a sustained fibrotic response in the heart that resulted in a distorted heart architecture and pump dysfunction. CFs are the largest cell population in the heart [33] ; however, CFs are still considered to play a secondary role in chronic heart failure. Due to the lack of inducible Cre-expressing lines that are effective for manipulating gene expression in mouse CFs, the regulatory mechanisms of pathological stress-induced fibrotic remodelling have not been fully elucidated. Several studies have revealed the central role of CFs in pathological fibrotic remodelling using the inducible Postn -Cre model [5] , [34] , [35] . As sources and targets of pathological stimuli, CFs coordinate mechanical and electrical signals among the cell populations of the heart [36] . Growth factors secreted by activated myofibroblasts directly induce cardiomyocyte hypertrophy in a paracrine-dependent manner [37] . Considering the critical role of CFs in cardiac fibrosis, identifying the key mediator of cardiac fibrosis would be of great clinical significance for designing novel therapeutics to prevent fibrotic remodelling. Recent studies have revealed that the IRX family of cardiac transcription factors is important in the normal development of the heart in rodents and humans [8] , [38] . Specifically, loss of IRX4, a member highly expressed in cardiomyocytes, causes cardiomyopathy characterized by cardiac hypertrophy and impaired contractile function [39] . Here, starting from the identification of fibrosis-related IRX members using rodent and human CFs, we found that IRX2 expression was upregulated in murine fibrotic hearts and failing human hearts. This pattern of upregulation was supported by results obtained with a mouse DCM model but challenged by a study reporting that IRX2 expression during the hypertrophic response was unchanged [40] . These incompatible results may be explained by the different phases and degrees of the fibrotic response between these reports. Moreover, we identified IRX2 as a CF-enriched transcription factor, implying a distinct role for IRX2 during the development of cardiac fibrosis. Irx2 -deficient mice do not display a notable phenotype in the heart structure or electrical conduction [41] . IRX2 was not essential for normal heart development, likely being functionally redundant with other IRX members. Our results provide the first indication for a role for IRX2 in regulating the pathophysiological process of cardiac fibrosis. In both our Ang II and transverse aortic constriction (TAC) models of fibrosis, we observed a reduction in fibrosis that was accompanied by an improvement in cardiac function in mice with CF- or myofibroblast-specific Irx2 depletion. Surprisingly, but not unexpectedly, this attenuated fibrotic response was not observed in mice with cardiomyocyte-specific Irx2 depletion, suggesting that IRX2 derived from CFs, not cardiomyocytes, plays a critical role in Ang II-induced fibrotic remodelling in mice. Most importantly, Irx2 mfTg mice demonstrated a pathological phenotype and deteriorated cardiac function upon Ang II infusion. Inconsistent with our findings, Wang and his colleagues observed that lentivirus injection-induced Irx2 knockdown prevented mice from Ang II-induced cardiac hypertrophy in mouse heart [42] . These incompatible results may be explained by the different manipulation of myocardial IRX2. Several studies have raised concerns that Col1α2-driven gene deletion was of limited value in deciphering the mechanism of cardiac fibrosis [43] , [44] . The use of Col1α2-driven Irx2 deletion didn’t compromise our main finding that IRX2 is a master regulator of pathological cardiac fibrosis. The limitation of Col1α2-driven IRX2 deletion was addressed with the use of Postn -Cre-mediated IRX2 deletion. Upon stimulation, CFs rapidly differentiate into myofibroblasts, which express the highly contractile protein α-SMA [45] , [46] . This conversion is a signature of an ongoing fibrotic response. Consistent with the fibrosis phenotype observed in vivo, fibroblast-to-myofibroblast transformation was significantly blocked after Irx2 loss of function but enhanced by Irx2 gain of function. Proliferation of activated CFs is another hallmark of fibrosis and plays an important role in the pro-fibrotic effects induced by Ang II [3] . In our study, IRX2 did not affect Ang II-induced CF proliferation, which was consistent with a previous report demonstrating that IRX2 promoted leukaemia cell differentiation without affecting cell proliferation [47] . IRX2 gain of function didn’t impact fibrotic phenotype basally, but deteriorated Ang II infusion-induced fibrotic phenotype, implying that there was a post-translational upstream switch for activating IRX2 transcription activation. Consistent with this hypothesis, Matsumoto et al reported that mitogen-activated protein kinase kinases 1, which was continually activated during fibrotic process, phosphorylated IRX2 protein to induce its activation in chick [13] . Deciphering the upstream regulation IRX2 would be of great translational significance. The limitation of our study is that whether IRX2 inhibition can reverse fibroblast-to-myofibroblast transformation remains unclear. This warrants further investigation. Identification of the fibrosis-promoting role of IRX2 raised another important question: what factors are responsible for IRX2-mediated cardiac fibrosis? There have been no reports describing the downstream targets of IRX2. We performed a bioinformatic intersection analysis between transcriptomic and ChIP-seq data and identified Egr1 as an IRX2 target. Our data showed that IRX2 could directly bind to the promoter of the Egr1 gene and promote its transcription in CFs. To the best of our knowledge, this is the first report describing the regulation of Egr1 by IRX2. Interestingly, Ang II-induced EGR1 expression was blocked by Irx2 depletion but enhanced by Irx2 gain of function. Given the critical role played by EGR1 in fibrosis, EGR1 modulation might be a key mechanism by which IRX2 promotes fibrotic remodelling in mice. This hypothesis was verified by our studies assessing genetic depletion of Egr1 , which rescued the pathological phenotypes observed in mice with myofibroblast-specific IRX2 overexpression. These data were in agreement with a report showing that Egr-1 deficiency protected against organ fibrosis in mice [48] . However, there sounds a different voice that global Egr1 knockout increased the number of fibrotic loci [49] . Egr1 depletion exacerbated, rather than attenuated, carbon tetrachloride-induced hepatic fibrosis [50] . These incompatible results suggested EGR1 played a context-dependent role in fibrogenesis, possibly determined by the injury onset and activated cell types. Accumulating evidence has demonstrated that the transcription factor EGR1 acts as an important mediator of fibroblast activation and the fibrotic response [29] . Herein, we also found that increased EGR1 expression directly induced fibroblast-to-myofibroblast transformation and regulated several fibrosis-related genes. The EGR1-dependent regulation of these fibrosis-related genes has been reported previously [29] , [51] . In our study, IRX2 regulated several pro-fibrotic factors in Ang II-infused CFs in an EGR1-dependent manner. The upregulation of TGF-β3 and PDGF members, as well as the activation of the Smad3 signalling pathway, contributed to the pathological phenotype observed in mice with myofibroblast-specific Irx2 overexpression. In our study, we also found that myofibroblast-specific Irx2 depletion, but not cardiomyocyte-specific Irx2 depletion, could attenuate cardiac hypertrophy, and improve cardiac systolic function. Growth factors and cytokines produced by CFs, were closely involved into the development of cardiac hypertrophy via paracrine-mediated cell-cell communications [37] . The decreased secretion of myofibroblasts-derived pro-hypertrophic factors (TGF-β, PDGF-A and PDGF-B) in mice with myofibroblast-specific Irx2 depletion in response to Ang II infusion might explain the improvement in cardiac hypertrophy and systolic function. In summary, this study identified IRX2 as a critical regulator of cardiac fibrosis via the transcriptional activation of EGR1. These observations advance our understanding of the mechanisms of pathological cardiac fibrosis. Study Design All animal studies were conducted in accordance with the guidelines for the Care and Use of Laboratory Animals published by the United States National Institutes of Health (NIH Publication, revised 2011) and the guidelines of the Animal Care and Use Committee of Renmin Hospital of Wuhan University. The objective of this study was to investigate the role of IRX2 in pathological cardiac fibrosis. The sample size of the animals was determined according to our previous study [52] . Investigators were blind to the animal experimental group. No samples were excluded from the analysis. Figure legends list the sample size, number of biological replicates, number of independent experiments. Animals and treatments Mice with a conditional knockout allele of Irx2 ( Irx2 fl/fl ) were acquired from Biocytogen Pharmaceuticals (Beijing, China). To achieve this knockout, the second and third exons were flanked by loxP sites, and thus, two single guide RNAs (sgRNA4 and sgRNA11) targeting the second and third exons were constructed. Purified Cas9 mRNA and two sgRNAs (sgRNA4: 5’-TGCCAAGACCCGCTCTGGCGGGG-3’;sgRNA11: 5’-GAAGAAAGACTACACCCACCAGG-3’) were then injected into zygotes, which were subsequently implanted into pseudopregnant mice. From 174 transferred zygotes, we identified one founder (#24) that possessed floxed second and third exons within the same allele. Successful generation of this conditional knockout allele was validated by touchdown PCR with the KOD-FX enzyme (#KFX-101, TOYOBO, Osaka, Japan) using the following Irx2 -specific primers: forward, 5’-GCATCAAGCTTGGTACCGATCAGAGCTCGTAGGCTGATTTCCCT-3’; and reverse, 5’-ACTTAATCGTGGAGGATGATGCAGTTAGTGAGGACAGGCTACAGC-3’. Tamoxifen-inducible Col1α2 -CreER mice (strain #029567) and injury-inducible Postn -Cre mice (Postn tm2.1(cre/Esr1*)Jmol , strain #029645) were purchased from The Jackson Laboratory (Bar Harbor, USA). Irx2 cfKO mice were bred by crossing Irx2 fl/fl mice with Col1α2 -Cre mice. To induce Cre recombinase expression in Irx2 cfKO mice, adult mice were intraperitoneally injected with tamoxifen (25 mg/kg per day, #T-5648, Sigma–Aldrich, St. Louis, USA) for five consecutive days. The dose of tamoxifen was selected according to our previous study [19] . After a 2-week washout period, IRX2 in isolated CFs was detected by western blotting. Injury-inducible conditional myofibroblast-specific Irx2 mfKO were bred by crossing the obtained Irx2 fl/fl mice with Postn -Cre mice. These mice were intraperitoneally injected with tamoxifen (25 mg/kg per day) for five consecutive days beginning from the first day of Ang II infusion and fed with a diet containing 400 mg/kg tamoxifen citrate (#130860, Envigo) from the first day of Ang II infusion until the time of sacrifice. Mice carrying the α-Mhc -MerCreMer construct (A1cf Tg(Myh6-cre/Esr1*)1Jmk , strain #005657) were obtained from The Jackson Laboratory; these mice were used in our previous studies [19] . Cardiomyocyte-specific Irx2 cmKO mice were generated by mating Irx2 fl/fl mice with α-Mhc -Cre mice. To further confirm the role of IRX2 in cardiac fibrosis, we used myofibroblast-specific Irx2 mfTg mice. Conditional transgenic founder mice expressing the Irx2 gene ( Irx2 Tg fl/fl ) were generated by Cyagen Biosciences Inc. (Guangzhou, China). The scheme for the construction of these mice is shown in Supplementary Fig. 6A . Successful generation of these conditional transgenic mice was validated by PCR with Irx2 -specific primers (forward, 5’-GATCCCCATCAAGCTGATCCG-3’; reverse, 5’-TACGGGTGGTAGCTGATGGC-3’) and internal control PCR primers (forward, 5’-GCAGAAGAGGACAGATACATTCAT-3’; reverse 5’-CCTACTGAAGAATCTATCCCACAG-3’). Injury-inducible Irx2 mfTg mice were bred by crossing Irx2 Tg fl/fl mice with Postn -Cre mice. These mice were intraperitoneally injected with tamoxifen (25 mg/kg per day) for five consecutive days beginning from the first day of Ang II infusion and fed with a diet containing 400 mg/kg tamoxifen citrate from the first day of Ang II infusion until the time of sacrifice. The transgenic leakiness of Irx2 mfTg mice was evaluated by evaluating IRX2 protein expression in the liver, lungs, kidneys, and heart. To verify the hypothesis that EGR1 mediates IRX2-induced pro-fibrotic effects, we investigated the role of EGR1 in IRX2-mediated cardiac fibrosis using Egr1 global knockout mice (strain #012924, The Jackson Laboratory). EGR1 deficiency was confirmed by western blotting. These mice were free access to water and food with five mice per cage. They were kept in a specific pathogen-free (SPF) condition with 20-25 °C temperature and 45-55% humidity on a regular 12 hour light/dark cycle. All animal experiments were performed in male mice to avoid possible shielding of estrogens. A cardiac fibrosis model was established by long-term Ang II infusion. Briefly, 8- to 10-week-old Irx2 cfKO or injury-inducible Irx2 mfKO mice, along with corresponding age-matched littermate control mice, were implanted with osmotic minipumps (ALZET; Durect Corp) containing Ang II (1,000 ng/kg/min, H1705, Bachem, Bubendorf, Switzerland) or the same volume of saline for 12 weeks in our and other studies [19] , [20] . These osmotic minipumps were implanted subcutaneously in mice under anaesthesia with 2% isoflurane. To test the hypothesis that Irx2 mfTg mice are more vulnerable to Ang II and exhibit accelerated development of cardiac dysfunction in response to Ang II infusion, Irx2 mfTg mice and age-matched littermate control mice were subjected to Ang II infusion for 4 weeks because 4 weeks of Ang II infusion can induce cardiac hypertrophy and fibrosis without altering the left ventricular EF [20] , [21] . Pressure overload is another well-studied mouse model of cardiac fibrosis. Briefly, thesse mice were anesthetized by intraperitoneal injections of 3% pentobarbital sodium, and the adequacy of anaesthesia was assessed by the pedal withdrawal reflex, breathing, and response to operation. The left chest was exposed by performing a ministernotomy, and the thoracic aorta was identified at the second intercostal space. Transverse aortic constriction was preformed with a 27-G needle using a 7-0 silk suture. After that, the needle was removed, and the thoracic cavity was closed. During the surgery, the body temperature was maintained by a warming pad [19] , [53] . Temgesic (0.1 mg/kg/day) was used to relieve postoperative pain. The adequacy of ligation was confirmed by validating increased blood flow velocity using Doppler echocardiogram. The mice in the sham groups underwent a similar procedure without ligation. Echocardiography was performed at 6 weeks after surgery. Mice were sacrificed by cervical dislocation at the end of these experiments. Blood pressure measurement and echocardiography Twelve weeks after Ang II infusion, the systolic blood pressure of conscious mice was measured by a non-invasive tail-cuff method. Transthoracic echocardiography was performed with a Vevo® 3100 high resolution Preclinical Imaging 496 System (FUJIFILM VisualSonics, Toronto, Canada) equipped with a 30-MHz linear ultrasound transducer [19] , [54] , [55] , and echocardiographic parameters were averaged from three to four cardiac cycles. During echocardiography, particular attention was given to avoid exerting excessive pressure on the chest of the mice anaesthetized with 2% isoflurane. Histological analysis and immunofluorescence staining Hearts were arrested in 10% KCl and fixed with 10% neutral formalin. After dehydration and embedding in paraffin, cardiac tissues were subsequently sectioned. Alexa Fluor™ 488 conjugate of wheat germ agglutinin (WGA, #W11261, Invitrogen, Carlsbad, USA) was used in order to measure cross-sectional area of cardiomyocytes. Sections were incubated with WGA (1:100) at 37 °C for 2 h. SlowFade TM Gold Antifade Mountant with DAPI (#S36939, Invitrogen) was used to stain nuclei. The value of cross-sectional area from each heart was averaged from more than 30 cells of an individual heart. These sections were then stained with picrosirius red (PSR) to evaluate the volume of fibrosis in the hearts. The value of fibrotic area was averaged from more than 10 fields from an individual heart. To determine the cellular location of IRX2 in hearts, sections were stained with anti-IRX2 (1:200, #AF0552, Affinity Biosciences, CA, USA), anti-cTnT (1:200, #ab8295, Abcam, Cambridge, UK) or anti-Col1 (1:200, #ab6308, Abcam) overnight, followed by an incubation with an Alexa Fluor 568-conjugated goat anti-rabbit IgG (H + L) cross-adsorbed secondary antibody (#A-11011, Invitrogen) and Alexa Fluor 488-conjugated goat anti-mouse IgG (H + L) cross-adsorbed secondary antibody for 1 h [19] . The specificity of the anti-IRX2 antibody from Affinity Biosciences was verified in conditional Irx2 -deficient mice or Irx2 -deficient CFs. To determine POSTN + /IRX2+ CFs, sections were stained with anti-IRX2 (1:200) and anti-POSTN (1:200, # 66491-1-Ig, Proteintech Group, Inc, Chicago, USA) overnight. The number of POSTN + /IRX2+ CFs was determined by investigators blinded to specific treatment. A minimum of 10 fields were analyzed every mouse and the average number of POSTN + /IRX2+ CFs for each sample was then calculated. To determine the subcellular location of IRX2, CFs were stained with anti-IRX2 at a dilution of 1:100 overnight, followed by an incubation with an Alexa Fluor 488-conjugated goat anti-rabbit IgG (H + L) highly cross-adsorbed secondary antibody (#A-11034, Invitrogen) for 1 h. To assess the expression of α-SMA, CFs were fixed with 4% formaldehyde, permeabilized in 0.1% Triton X-100 and stained with anti-α-SMA (#ab7817, Abcam) at a dilution of 1:200 overnight, followed by an incubation with an Alexa Fluor 488-conjugated goat anti-mouse secondary antibody (#A11017, Invitrogen) for 1 h. SlowFade TM Gold Antifade Mountant with DAPI (#S36939, Invitrogen) was used to stain nuclei. To assess the area of cardiomyocytes in vitro, cardiomyocytes were stained with anti-α-actinin (#05-384, Merck Millipore) at a dilution of 1:200 overnight, followed by an incubation with an Alexa Fluor 568-conjugated goat anti-mouse IgG (H + L) cross-adsorbed secondary antibody (#A-11004, Invitrogen). Slides were examined in a blinded manner, and the results generated with Image-Pro Plus 6.0 (Media Cybernetics, Silver Springs, MD, USA) were confirmed independently by two authors. Human heart samples Human heart samples have been used in previous reports [19] , [56] . Human fibrotic heart samples were taken from the left ventricle of DCM patients undergoing cardiac transplantation. Control heart samples were obtained from normal heart donors whose hearts were not suitable for transplantation for non-cardiac reasons. Detailed information for the donors and patients with DCM was previously presented [56] . For donor group, 2 females and 4 males were included. For DCM group, 2 females and 5 males were included. All donors and patients with DCM have signed written informed consent, and all human experiments were conducted in accordance with the Declaration of Helsinki and approved by our Institutional Review Board (Renmin Hospital of Wuhan University Review Board). Western blotting and quantitative real-time PCR Total protein was extracted from heart tissues with lysis buffer containing a protease inhibitor cocktail (#11852700, Roche, Basel, Switzerland) and phosphatase inhibitor (#04906837001, Roche). Protein concentrations were determined with a BCA assay kit (#23227, Invitrogen). The proteins were electrophoresed by SDS–PAGE (10% gel) [19] , [54] , [57] and transferred to polyvinylidene fluoride membranes (#IPFL00010, Millipore, MA, USA). After blocking with 5% non-fat milk for 2 h, the membranes were incubated with the following primary antibodies overnight at 4 °C: anti-IRX2 (1:500, #AF0552, Affinity Biosciences), anti- CTGF (1:500, #ab6992, Abcam), anti-EGR1 (1:1000, #55117-1-AP, Proteintech, Manchester, UK), anti-Smad3 (1:500, #9513 S, Cell Signaling Technology, Danvers, MA, USA), anti-phosphorylated Smad3 (p-Smad3, 1:500, #8769, Cell Signaling Technology), and anti-GAPDH (1:2000, #2118, Cell Signaling Technology), followed by incubation with horseradish peroxidase-conjugated secondary antibodies at room temperature for 1 h. Blots were visualized with an enhanced chemiluminescence kit (#1705061, Bio–Rad Laboratories, Hercules, USA) and analysed using Image J software (Bio-Rad, Hercules, CA, USA). 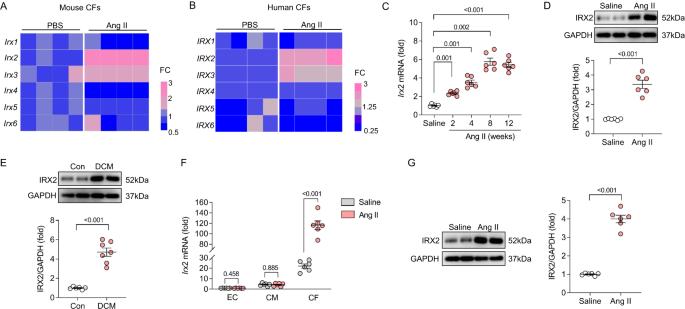Total RNA was extracted from frozen samples with TRIzol reagent (#15596018, Invitrogen). Total mRNA isolated from heart samples was reverse transcribed into complementary DNA (cDNA) with a Transcriptor First Strand cDNA Synthesis Kit (#04896866001, Roche, Basel, Switzerland). Fig. 1: IRX2 expression was increased in fibrotic hearts. ARelative mRNA levels of 6Irxfamily members in adult mouse cardiac fibroblasts (CFs) after angiotensin II (Ang II) treatment for 24 h (n= 5).BRelative mRNA levels of 6IRXfamily members in human CFs after Ang II treatment for 24 h (n= 5).CIrx2mRNA levels in the heart after Ang II infusion by an osmotic minipump (n= 6).DRepresentative western blots and statistical analysis of IRX2 expression in the heart after Ang II infusion for 12 weeks (n= 6).ERepresentative western blots and statistical analysis of IRX2 expression in heart samples obtained from patients with dilated cardiomyopathy (DCM) and control (Con) donors (Con,n= 6; DCM,n= 7).FIrx2mRNA levels in endothelial cells (ECs), cardiomyocytes (CMs) and CFs isolated from hearts infused with Ang II for 12 weeks (n= 6).GRepresentative western blots and quantification of IRX2 protein expression in CFs isolated from hearts infused with Ang II for 12 weeks (n= 6). Data are shown as the mean ± SEM, and analysed using an unpaired two-tailed Student′sttest. For the analysis in (C), one-way ANOVA with Tamhane’s T2 test was conducted. Source data are provided as a Source Data file. Reactions were quantified with LightCycler 480 SYBR Green 1 Master Mix (#04707516001, Roche) and appropriate primers (Supplementary Table 1 ). mRNA levels were normalized to those of Gapdh . Cell culture and treatment Adult mouse CFs were isolated as described previously [5] , [20] , [35] . Briefly, adult mice (6 to 8 weeks old) were anaesthetized with 2% isoflurane, and the hearts were excised and mounted on a Langendorff apparatus. After washing away the blood with Hanks’ Balanced Salt Solution (#24020117, Gibco, Grand Island, NY, USA), the hearts were perfused with hyaluronidase and collagenase II (2 mg/mL, #LS004176, Worthington, Lakewood, USA) for 25 min. After digestion, CFs were purified by removing other cells via a differential attachment technique. CFs were then cultured in Dulbecco’s modified Eagle’s medium (DMEM)/F12 (#51445 C, Gibco) supplemented with 10% FBS for 48 h. Then, the culture medium was replaced with serum-free DMEM/F12 for 12 h to synchronize the cells before experiments. After that, the CFs were treated with Ang II (1 μmol/l) for 24 h to mimic a fibrotic phenotype. To deplete IRX2 proteins, CFs isolated from IRX2 fl/fl mice were infected with an adenovirus carrying Cre or a control (Con) for 4 h at a multiplicity of infection of 50 and then treated with Ang II for 24 h. To further confirm IRX2 deficiency in the fibrotic phenotype, CFs isolated from wild-type (WT) mice were infected with adenoviral genome particles carrying shRNAs against Irx2 . The targeting sequences were as follows: 5’-TGGCCATTATCACCAAGATGACC-3’ (sh Irx2 #1), 5’-GGCTCTGAGTGTAAGGACAAGTTTG-3’ (sh Irx2 #2), and CATTGCTGGTTATACAATCTCTGTT (sh Irx2 #3). To further assess the role of IRX2 in the fibrotic response, CFs were infected with an adenovirus carrying Irx2 or Gfp for 4 h at a multiplicity of infection of 50. shRNA targeting mouse Egr1 (sequence: 5’-GCTGCTTCATCGTCTTCCTCT-3’) was used to further clarify the role of EGR1 in the IRX2-mediated fibrotic response in vitro. In addition, CFs were isolated from Egr1 -knockout mice and WT mice and infected with an adenovirus carrying Irx2 . Then, the cells were harvested to evaluate the role of EGR1 in the IRX2-mediated fibrotic response. CFs in the first and second passages were used in our studies. All the adenoviral vectors and shRNAs were provided by Hanbio Biotechnology Co., Ltd. (Shanghai, China). Normal human CFs were provided by Cell Applications Inc. (San Diego, CA). These human CFs were negative for contamination with several viruses, bacteria, and fungi. Human CFs were maintained in DMEM/F12 containing 10% FBS for 48 h and then infected with an adenovirus carrying IRX2 for 4 h at a multiplicity of infection of 50. To verify the hypothesis that EGR1 is responsible for the fibrotic effects of IRX2, Egr1 expression in human CFs was knocked down with an shRNA targeting human EGR1 (sequence: 5’-CCAUGGACAACUACCCUAATT-3’). 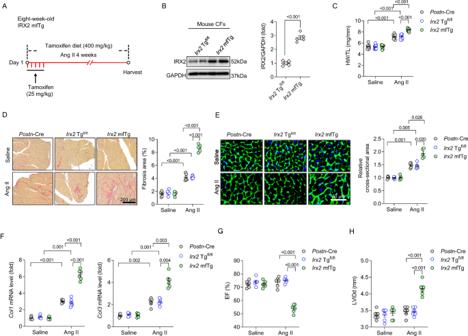Fig. 4: Conditional myofibroblast-specificIrx2overexpression promoted angiotensin II (Ang II)-induced fibrotic remodelling in mice. AConditional myofibroblast-specificIrx2-overexpressing mice (Irx2mfTg) were bred by crossing conditional transgenic mice expressing theIrx2gene (Irx2Tgfl/fl) withPostn-Cre mice.Irx2mfTg mice and their littermate controls were subjected to Ang II infusion for 4 weeks.BRepresentative western blots and statistical analysis of IRX2 protein expression in CFs isolated fromIrx2mfTg mice and littermate controls after Ang II infusion for 4 weeks (n= 5).CHeart weight to tibia length (HW/TL) ratio (n= 12 mice for all six groups).DCardiac fibrosis was determined by picrosirius red staining inIrx2mfTg mice after Ang II infusion (n= 5).ECell area of cardiomyocytes was determined with wheat germ agglutinin (WGA) staining inIrx2mfTg and littermate controls after Ang II infusion (n= 5).FRelative mRNA levels ofCol1andCol3were detected in the hearts ofIrx2mfTg mice and their controls (n= 6).G,HEjection fraction (EF) (G) and left ventricular end-diastolic dimension (LVIDd) (H) were detected in these groups (n= 6). The data were compared by one-way ANOVA. Data are shown as the mean ± SEM, and analysed using one-way ANOVA followed by Tukey post hoc test (C–DandG–H) or Tamhane’s T2 test (E–F). For the analysis in (B), an unpaired two-tailed Student′sttest was conducted. Source data are provided as a Source Data file. After Ang II stimulation for 24 h, the cells were harvested for the detection of several fibrotic markers. Neonatal rat cardiomyocytes (NRCMs) were isolated and cultured as described previously [56] , [57] . Briefly, hearts were quickly excised from neonatal Sprague–Dawley rats (1 to 3 days old) under sterile conditions and washed with DMEM/F12 3 times. After that, the atria and aorta were discarded, and the ventricles were minced into 1- to 2-mm pieces and digested with D-Hanks containing 0.125% trypsin (#25200, Gibco) for 20 min (5 min each time, 4 times) at 37 °C. The cells were then centrifuged at 250 g for 5 min, and the pellet was resuspended in DMEM/F12 containing 15% FBS. CFs were separated via a differential attachment technique. After that, NRCMs were plated in 35-mm dishes coated with gelatine. Bromodeoxyuridine (0.1 mmol/l) was used to prevent neonatal fibroblast contamination. To evaluate the crosstalk between CFs and cardiomyocytes, CFs were isolated from Irx2 cfKO mice and Irx2 fl/fl mice and then stimulated with Ang II for another 24 h to induce a fibrotic phenotype. Then, conditioned medium from these myofibroblasts was collected and used to treat NRCMs in the absence or presence of Ang II for another 24 h. After that, the cell area of cardiomyocytes was detected by immunofluorescence staining. Cardiac endothelial cells were isolated from adult mice using CD31 microbeads (Miltenyi Biotec) [19] . Analysis of cardiac fibroblast proliferation CFs isolated from Irx2 fl/fl mice were infected with an adenovirus carrying Cre or a control for 4 h. Twenty-four hours after infection, the CFs were cultured in DMEM/F12 with or without 5% FBS for 3 days. In addition, Irx2 fl/fl CFs were infected with an adenovirus carrying Cre and thereafter subjected to Ang II treatment for 3 days. CF proliferation was examined by an MTT assay. RNA-seq library preparation, sequencing and analysis CFs were infected with an adenovirus carrying Irx2 or Gfp and then subjected to Ang II stimulation for 24 h. After that, total RNA was extracted, and RNA degradation and potential contamination were determined with 1% agarose gels. RNA purity was determined with a NanoPhotometer® spectrophotometer (IMPLEN, CA, USA). The RNA concentration was measured with a Qubit® RNA Assay Kit on a Qubit® 2.0 Fluorometer (Life Technologies, CA, USA). RNA integrity was detected using an RNA Nano 6000 Assay Kit for the Bioanalyzer 2100 system (Agilent Technologies, CA, USA). Library construction was performed with a NEBNext® UltraTM RNA Library Prep Kit Illumina® (NEB, USA) with 3 µg RNA per sample following the manufacturer’s recommendations. Library quality was evaluated with an Agilent Bioanalyzer 2100 system. After cluster generation with TruSeq PE Cluster Kit v3-cBot-HS (Illumina), the library preparations were sequenced on an Illumina HiSeq platform, and paired-end reads were generated. Three independent biological replicate samples were sequenced for each group. After removing low-quality reads with FASTX-Toolkit, the high-quality clean data were aligned to a mouse genome (mm10) with HISAT2. Differentially expressed gene (DEG) analysis between the two groups was conducted with the DESeq2 R package. RNA-seq and subsequent analyses were performed by Novogene (Beijing, China). ChIP, ChIP-seq and ChIP-PCR Human CFs were infected with an adenovirus carrying IRX2 for 4 h and then subjected to Ang II stimulation for 24 h. After that, the cells were cross-linked with 1% formaldehyde for 10 min. Then, glycine (0.125 mol/l) was added to terminate the cross-linking reaction. The cross-linked cells were harvested with lysis buffer containing a complete protease inhibitor mixture, and the nuclei were collected by centrifugation at 2000 g for 5 min. After that, the nuclei were further treated with nuclear lysis buffer and sonicated (15 times, 30 s on/off). Precipitation was performed with an anti-IRX2 antibody (#PCRP-IRX2-1B7, Developmental Studies Hybridoma Bank, Houston, USA; or #PCRP-IRX2-1C1, Developmental Studies Hybridoma Bank) incubated overnight at 4 °C. The DNA–protein complexes were used for immunoblot analysis to verify the precipitation of IRX2. After confirmation, DNA was purified with a QIAquick PCR purification kit (#28104, Qiagen) after reversing the cross-linking and performing protease K digestion. Sequencing libraries were prepared by using a VAHTS Universal DNA Library Prep Kit for Illumina V3 (#ND607, Vazyme). The library products corresponding to 200-500 bps were enriched, quantified and finally sequenced on a NovaSeq 6000 sequencer (Illumina) with the PE150 model. ChIP-seq with input DNA and ChIP DNA was performed by Seqhealth (Wuhan, China). Raw reads were processed to include only high-quality reads using Trimmomatic. Clean data were compared to a human genome (hg19) using STAR software (version 2.5.3a). Only uniquely aligned reads were retained for subsequent bioinformatic analysis. Read distribution analysis was performed with RSeQC (version 2.6). To identify a significant binding site of IRX2, peak calling was performed with MACS2 (version 2.2.7.1), with the input used as the control. Peaks with P values < 0.01 were kept for further analyses. Peak annotation was performed with BEDTools (Version v2.25.0). Motif analysis was performed with Homer (version 4.10). ChIP-PCR was performed using primers (forward 5’-CCCTGGATGACAGCGATAGAA-3’; reverse 5’-CAAATAAGGGTTGTTCCGGCG-3’) spanning the IRX2 binding site in the Egr1 promoter. Luciferase reporter gene assay To evaluate the regulation of EGR1 by IRX2, an Egr1 promoter clone (chr18 + :35019534-35021123) was obtained from iGene Biotechnology Co., Ltd. (#MPRM16005, Guangzhou, China). This promoter clone was inserted into a pGL3 promoter luciferase vector ( Egr1 -Luc). CFs isolated from WT mice were cultured for 48 h and then infected with an adenovirus carrying Irx2 for 4 h. After infection, the CFs were electrotransfected with Egr1 -Luc (0.03 μg) with the Neon® Transfection System (pulse voltage: 1700 V, pulse width: 20 ms) and treated with Ang II. After Ang II incubation for 24 h, the cells were harvested, and luciferase activity was measured using dual-luciferase assay kits (Promega, Madison, USA). The Egr1 promoter 1×mutant or 2×mutant were also generated by one-step PCR mutagenesis to delete one (ACAGGTGG) or two IRX2 binding sites (ACAGGTGG and ACAGTGT). To confirm that IRX2 promoted fibroblast activation directly through interaction with the Egr1 promoter, Irx2 -overexpressed CFs were infected with an adenovirus carrying mutated Egr1 promoter with two IRX2 binding sites deletion. Statistical analysis Results are expressed as the mean ± SEM. We used the Shapiro–Wilk test to evaluate data normality. Comparisons among more than two groups were performed by one-way ANOVA followed by the post hoc Tukey test when the data had a normal distribution and ANOVA found no variance in homogeneity; otherwise, Tamhane’s T2 post hoc test was used (SPSS 26.0, SPSS Inc., Chicago, IL). Comparisons between two groups were performed using an unpaired Student’s t test. Repeated-measures ANOVA was performed to compare differences among groups over time. No samples were excluded from the analysis. 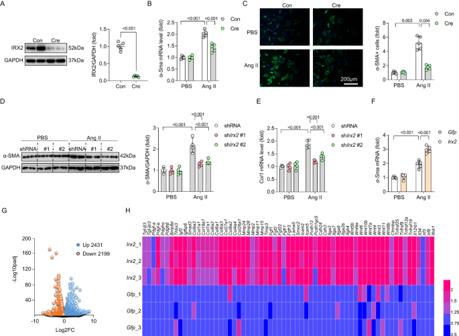Fig. 5: IRX2 is essential for fibroblast to myofibroblast transformation. AAdult cardiac fibroblasts (CFs) were isolated fromIrx2fl/flmice and infected with an adenoviral vector carrying Cre to depleteIrx2. After 24 h of transfection, IRX2 protein expression was detected in CFs (n= 5).BRelative mRNA level ofα-SmainIrx2-depleted adult mouse CFs (n= 5).CRepresentative images and quantification of α-SMA (green) in Cre-infectedIrx2fl/flCFs in response to Ang II incubation for 24 h. Nuclei are stained with DAPI (blue). (n= 5, for each group, 50-60 fields were counted).DCFs were isolated from wild-type mice and then transfected with shRNAs targetingIrx2. After 24 h of transfection, the cells were subjected to Ang II treatment for 24 h to induce a fibrotic phenotype. After that, the cells were harvested for the detection of α-SMA with western blotting (n= 4).ERelative mRNA level ofCol1in IRX2-deficient CFs after Ang II incubation for 24 h (n= 4).FCFs were isolated from wild-type mice and then overexpressedIrx2with an adenovirus vector, after which they were subjected to Ang II treatment for 24 h. The relative mRNA level ofα-Smawas detected to reflect fibroblast to myofibroblast transformation (n= 5).GCFs were isolated from wild-type mice and then overexpressedIrx2with an adenovirus vector, after which they were subjected to Ang II treatment for 24 h. Total RNA was extracted, and RNA sequencing was performed. Volcano plots indicating the differentially expressed genes (DEGs) inIrx2-overexpressing CFs relative to controls after Ang II administration for 24 h.HHeatmap of several differentially expressed genes inIrx2-overexpressing CFs relative to controls after Ang II infusion. Data are shown as the mean ± SEM, and analysed using one-way ANOVA followed by Tukey post hoc test (BandD–F) or Tamhane’s T2 test (C). For the analysis in (A), an unpaired two-tailed Student′sttest was conducted. Source data are provided as a Source Data file. Statistical significance was assigned at p < 0.05. 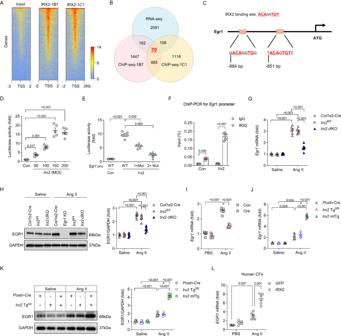Fig. 6: EGR1 was identified as a direct downstream target gene of IRX2 in cardiac fibroblasts that regulates the angiotensin II (Ang II)-induced fibrotic response. ACFs were infected with an adenovirus carryingIRX2and then subjected to Ang II stimulation for 24 h. ChIP-seq was performed with two anti-IRX2 antibodies (IRX2-1B7 and IRX2-1C1). Similar spatial distributions of IRX2 peaks were identified by the two anti-IRX2 antibodies.BIRX2-regulated genes identified in the ChIP-seq data (bottom) were overlaid with upregulated differentially expressed genes revealed by RNA-seq (top). With this strategy, 70 genes were identified.CTwo IRX2 binding sites were identified in the ChIP-seq peak distributed in the promoter site ofEgr1.DTheEgr1promoter was stimulated by IRX2 overexpression.Egr1promoter activity was measured by a luciferase assay uponIrx2overexpression in CFs isolated from wild-type mice (n= 5 for each group).EThe mutant (Mut) promoters (pro) deleting IRX2 binding sites cannot be stimulated byIrx2overexpression (n= 5 for each group).FIndependent ChIP-PCR was performed withIrx2-overexpressing CFs to verify IRX2 binding to the promoter ofEgr1(n= 5).G–HEgr1mRNA and EGR1 protein expression in CFs isolated fromIrx2cfKO mice and littermate controls with or without Ang II infusion for 12 weeks (n= 6).IEgr1mRNA levels were detected in CFs withIrx2deficiency caused by Cre expression (n= 5).J–KEgr1mRNA and EGR1 protein expression in CFs isolated fromIrx2mfTg mice and littermate controls with or without Ang II infusion for 4 weeks (n= 6).LEgr1mRNA level inIrx2-overexpressing human CFs after Ang II treatment for 24 h (n= 6). Data are shown as the mean ± SEM, and analysed using one-way ANOVA followed by Tukey post hoc test (H,IandK) or Tamhane’s T2 test (D–G,JandL). Source data are provided as a Source Data file. 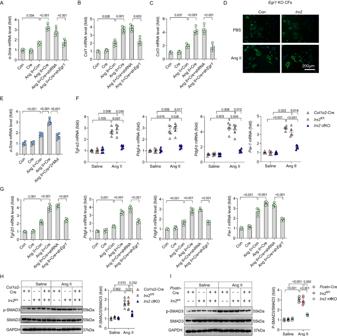Fig. 7: EGR1 was responsible for the IRX2-promoted fibrotic response in angiotensin II (Ang II)-treated cardiac fibroblasts. A–CCardiac fibroblasts (CFs) were isolated fromIrx2Tgfl/flmice and infected with an adenovirus carrying Cre to overexpressIrx2. After that,Egr1expression was knocked down, and the CFs were subjected to Ang II treatment for 24 h. After that, the cells were harvested to detect the mRNA levels ofα-Sma(A),Col1(B) andCol3(C) (n= 5).DRepresentative images of α-SMA (green) in CFs isolated fromEgr1-knockout mice after Ang II treatment for 24 h. Nuclei were stained with DAPI (blue) (n= 5, for each experiment, 50-60 fields were counted).ERelative mRNA levels ofα-Smain the indicated groups (n= 5).FRelative mRNA levels of fibrosis-related genes in CFs isolated fromIrx2cfKO mice and littermate controls with or without Ang II infusion for 12 weeks (n= 5).GCFs were isolated fromIrx2Tgfl/flmice and infected with an adenovirus carrying Cre to overexpressIrx2. After that,Egr1expression was knocked down, and the CFs were subjected to Ang II treatment for 24 h. After that, the cells were harvested to detect the mRNA levels of fibrosis-related genes (n= 5).H,IWestern blot analysis was performed to analyse the phosphorylation of Smad3 in CFs isolated fromIrx2cfKO orIrx2mfKO mice and corresponding littermate controls with or without Ang II infusion for 12 weeks (n= 6). Data are shown as the mean ± SEM, and analysed using one-way ANOVA followed by Tukey post hoc test (A,C,EandG) or Tamhane’s T2 test (B,F,HandI). Source data are provided as a Source Data file. 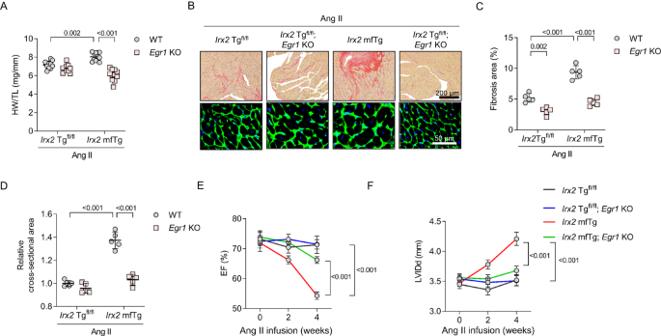Fig. 8: Genetic depletion ofEgr1attenuated fibrotic remodelling in mice with conditional myofibroblast-specificIrx2overexpression after angiotensin II (Ang II) infusion. Conditional myofibroblast-specificIrx2-overexpressing mice (Irx2mfTg) were bred withEgr1global knockout mice or wild type (WT). The resulting mouse line and littermate controls were subjected to Ang II infusion for 4 weeks.AHeart weight-to-tibia length (HW/TL) ratio (n= 10 mice,Irx2Tgfl/fl+ WT+Ang II;n= 10 mice,Irx2Tgfl/fl+Egr1KO+Ang II;n= 11 mice,Irx2mfTg+WT+Ang II;n= 11 mice,Irx2mfTg+Egr1KO+Ang II).BHistological staining showed cardiomyocyte enlargement and cardiac fibrosis after Ang II infusion (n= 5).CCardiac fibrosis was determined by picrosirius red staining after Ang II infusion (n= 5).DThe cell area of cardiomyocytes was determined with wheat germ agglutinin (WGA) staining after Ang II infusion (n= 5).E,FThe ejection fraction (EF) (E) and left ventricular end-diastolic dimension (LVIDd) (F) were detected in these groups (n= 6). Data are shown as the mean ± SEM, and analyzed using one-way ANOVA followed by Tukey post hoc test (A,C, andD). For the analysis in (E,F), repeated measures ANOVA was conducted. Source data are provided as a Source Data file. Reporting summary Further information on research design is available in the Nature Portfolio Reporting Summary linked to this article.